Photoelectrocatalytic C–H halogenation over an oxygen vacancy-rich TiO2photoanode Photoelectrochemical cells are emerging as powerful tools for organic synthesis. However, they have rarely been explored for C–H halogenation to produce organic halides of industrial and medicinal importance. Here we report a photoelectrocatalytic strategy for C–H halogenation using an oxygen-vacancy-rich TiO 2 photoanode with NaX (X=Cl − , Br − , I − ). Under illumination, the photogenerated holes in TiO 2 oxidize the halide ions to corresponding radicals or X 2 , which then react with the substrates to yield organic halides. The PEC C–H halogenation strategy exhibits broad substrate scope, including arenes, heteroarenes, nonpolar cycloalkanes, and aliphatic hydrocarbons. Experimental and theoretical data reveal that the oxygen vacancy on TiO 2 facilitates the photo-induced carriers separation efficiency and more importantly, promotes halide ions adsorption with intermediary strength and hence increases the activity. Moreover, we designed a self-powered PEC system and directly utilised seawater as both the electrolyte and chloride ions source, attaining chlorocyclohexane productivity of 412 µmol h −1 coupled with H 2 productivity of 9.2 mL h −1 , thus achieving a promising way to use solar for upcycling halogen in ocean resource into valuable organic halides. Photoelectrochemical (PEC) technology is regarded as an environmentally benign route for H 2 production via water splitting. In a typical PEC cell for water splitting, the photoexcited electrons from the photoanode are transferred to the photocathode to drive H 2 O reduction to produce H 2 , and the photogenerated holes left on the photoanode are employed for the oxidation of H 2 O to O 2 (Fig. 1a ) [1] , [2] . However, the reaction efficiency is always hindered by the energetically and kinetically demanding O 2 evolution reaction (OER) [3] , [4] . In recent years, PEC works have circumvented this limitation by introducing organic molecules oxidation reactions which are energetically more favorable than OER, making it an attractive strategy that promotes H 2 production rate and simultaneously produces value-added chemicals from cheap organic compounds [5] , [6] . However, the reaction variety is limited to the oxidation of simple alcohol substrates and oxygenated biomass feedstocks [7] , [8] , [9] , [10] , [11] such as 5-Hydroxymethylfurfural (HMF) [7] , [8] and benzyl alcohol [11] . Recently, significant developments have been made on C–H functionalization in PEC cell system, achieving the construction of carbon–heteroatom bonds to produce high value-added chemicals over the photoanode at mild conditions (Fig. 1b ) [12] , [13] , [14] . For instance, Wu and co-workers successfully realized the P–H/C–H cross-coupling to construct C–P bond via a PEC process, which showed good functional-group tolerance, broad substrate scope and high yield [12] . Hu and co-workers creatively developed an efficient PEC strategy to achieve non-directed arene C–H animation with high ortho selectivity over a hematite photoanode [13] . Despite these progresses, there is only a handful of carbon–heteroatom bonds that can be constructed in PEC cell system, involving C–N, C–O, and C–P bonds [14] . Therefore, the development of efficient PEC strategy for C–H functionalization to construct more types of carbon–heteroatom bonds is yet to be explored and highly desirable. Fig. 1: PEC cells. a PEC water oxidation coupled with H 2 production. b PEC C–H functionalization coupled with H 2 production. CB conduction band, VB valence band. Full size image Organic halides are a family of important fine chemicals that have wide applications in various branches of chemistry (e.g., medicines, dyestuffs, agrochemicals, etc), as well as in electronic and metalworking industries [15] . The conventional synthesis methods involve thermal homogeneous or heterogeneous catalytic processes (Fig. 2a ) [16] , [17] , [18] , [19] , [20] , [21] , [22] , [23] . Although efficient and well-reported in literatures, these methods have limitations that hinder the production in a sustainable manner, such as the use of hazardous and expensive halogenation reagents (such as dihalogen or N -halogensuccinimide) [16] , [17] , the need of metal salts as the catalysts (e.g., CoX 2 , CuX 2 , LiX, etc) that are difficult to be separated and reused [18] , [19] , the need of external oxidants (e.g., O 2 , 2KHSO 5 ·KHSO 4 ·K 2 SO 4 , AgSbF 6 , etc) [20] , [21] and elevated temperature [22] , [23] . Very recently, Lei and co-workers reported an electrochemical oxidation method for C–H halogenation with HX/NaX, showing broad substrate scope and high efficiency [24] (Fig. 2b ). Nevertheless, this process still needs large external bias (>2.5 V vs. RHE), and organic solvent (e.g., MeCN, DMF) and electrolyte (e.g., n Bu 4 NBF 4 ) are required for optimum reaction conditions. Compared with electrocatalytic method, photoelectrocatalytic method is expected to reduce the applied external bias, therefore saving electricity and potentially suppressing side reactions that may proceed under high applied voltage. It is reported that halogenation reaction is a typical free radical-mediated process, in which the halogen radicals react with the substrates containing C–H bonds to yield organic halides [16] , [18] , [25] . Thus, we speculate that halogenation reaction can proceed in the PEC cell with halogen ions if the photogenerated holes in the valence band (VB) of photoanodes is more positive than the oxidation potential of the halogen ions to halogen radicals (Fig. 2c ). However, direct C–H halogenation has never been explored in PEC cells. Fig. 2: C–H halogenation. a Thermocatalytic process. b Electrocatalytic process. c Photoelectrocatalytic process (this work). Full size image In this work, we report a photoelectrocatalytic strategy for C–H halogenation with NaX (X=Cl − , Br − , I − ) over an oxygen-vacancy-rich TiO 2 photoanode, producing high value-added organic halides coupled with cathodic H 2 production (Fig. 2c ). The NaX aqueous solution (pH = 7) is used as both the electrolyte and halide source. Specifically, we achieve monochlorination of cyclohexane to chlorocyclohexane in 92.5% selectivity with yield of 0.064 mmol cm −2 h −1 . Experimental integrated with spin-polarized density functional theory (DFT) studies reveal that the PEC chlorination of cyclohexane mainly follows a free radical chain reaction process, in which the chlorine radicals and Cl 2 are generated through the activation of halogen ions catalyzed by the photogeneated holes over TiO 2 . The strategy exhibits broad substrate scope for arenes, heteroarenes, nonpolar cycloalkanes, and aliphatic hydrocarbons. Moreover, both experimental and theoretical results indicate that the oxygen vacancies on TiO 2 help enhance the adsorption of halogen ion and thus their enrichment in local environment, together with the enhanced photo-induced carriers separation efficiency. Finally, we design a self-powered PEC system and directly utilized seawater as the electrolyte and the Cl − source, attaining chlorocyclohexane productivity of 412 µmol h −1 coupled with H 2 productivity of 9.2 mL h −1 . As a result, we achieve a promising way to use solar for upcycling halogen in ocean resource into valuable organic halides. Screening and optimization of photoanodes Cyclohexane was selected as the model substrate for PEC chlorination reaction. The PEC tests were performed in a three-electrode configuration in a H-type quartz cell, and Pt foil was used as the cathode and Ag/AgCl electrode as the reference electrode. A NaCl aqueous solution (0.5 M, pH = 7) was used as both the electrolyte and chlorine source. Several typical semiconductors (TiO 2 , WO 3 , BiVO 4 , and ZnO) were synthesised and screened as the photoanode (the synthesis methods and structural characterisations see experimental section and Supplementary Fig. 1 ). Linear sweep voltammetry (LSV) curves in Supplementary Fig. 2 show that TiO 2 exhibits higher photocurrent density compared to other semiconductors in a 0.5 M NaCl electrolyte containing 18.8 mmol cyclohexane under AM 1.5G irradiation (that is 100 mW cm −2 ), and achieves higher cyclohexane conversion rate of 16 µmol cm −2 h −1 at 1.6 V vs. RHE (Fig. 3a ). The gas chromatography-mass spectrometry (GC-MS, Supplementary Fig. 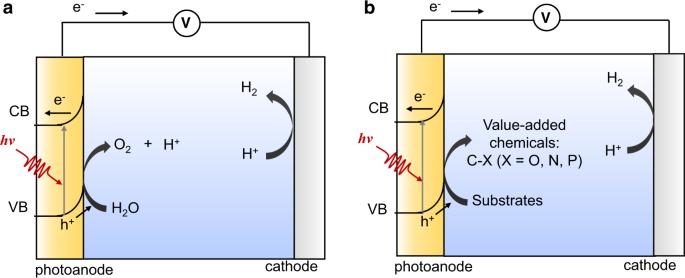Fig. 1: PEC cells. aPEC water oxidation coupled with H2production.bPEC C–H functionalization coupled with H2production. CB conduction band, VB valence band. 3 and Supplementary Table 1 ) show that chlorocyclohexane (2a) is the main product over different photoanodes with selectivity in the range of 82.3–88.0% and FE of 56.8–68.5%. This indicates the efficacy of PEC strategy for chlorination reaction, although the selectivity of chlorocyclohexane requires further improvement. We notice that the byproducts include cyclohexanol (2b), cyclohexanone (2c), bicyclohexyl (2d) and cyclohexene (2e) with much lower selectivity. Among them, cyclohexanol and cyclohexanone are likely attributed to the oxidation of cyclohexane by hydroxyl radicals from H 2 O [26] , [27] , cyclohexene is due to the dehydration of cyclohexanol, and bicyclohexyl may come from the recombination of cyclohexane radical [18] . Due to the higher catalytic performance of TiO 2 in PEC chlorination of cyclohexane, we focus on it for further study. Fig. 3: Cyclohexane chlorination performance via PEC. a Photoelectrocatalytic conversion rate of cyclohexane and corresponding products selectivity over typical semiconductors. b Photoelectrocatalytic conversion rate of cyclohexane and corresponding products selectivity over TiO 2 -O v - T ( T represents the temperatures, 200, 350, 400, and 450 °C) photoanodes. c Stability test of TiO 2 -O v -400 photoanode for the chlorination of cyclohexane for 255 h in batch reaction (85 batches). The reaction was carried out in a batch reaction in 0.5 M NaCl with 18.8 mmol cyclohexane at 1.6 V vs. RHE under AM 1.5G, 100 mW cm −2 illumination, with 3 h for one batch. The spent TiO 2 -O v -400 photoanode was washed by deionized water and dried under vacuum for the next batch reaction. The error bars represent the relative deviation, which is within 5%. The curves in each figure are guides to the eye. Full size image Previous reports reveal that introducing oxygen vacancy can effectively enhance the photo-induced charge separation and visible light absorption performances for TiO 2 photoanode [28] . We thus explored the effect of oxygen vacancy on PEC chlorination reaction over the TiO 2 photoanode. The oxygen vacancy was generated through treating the pristine TiO 2 photoanode with H 2 under different temperatures. The treated samples are denoted as TiO 2 -O v - T ( T represents the temperatures, 200, 350, 400, and 450 °C were used; Supplementary Fig. 4 ). The formation of oxygen vacancy was identified by X-ray photoelectron spectroscopy (XPS; Supplementary Fig. 5 ), in which the O 1 s XPS spectra of all the TiO 2 -O v - T samples show a typical oxygen adsorption peak at the bonding energy of 531.4 eV, which are assigned to the oxygen vacancy [28] , [29] . 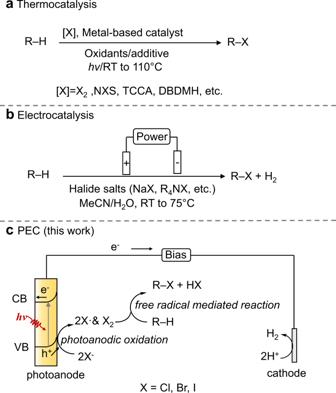Fig. 2: C–H halogenation. aThermocatalytic process.bElectrocatalytic process.cPhotoelectrocatalytic process (this work). The corresponding peak intensity was enhanced with the increase of H 2 treatment temperature, an indicative of the increased oxygen vacancy concentration (Supplementary Table 2 ), consistent with the previous reports [29] . The as-prepared TiO 2 -O v - T samples were then tested for PEC chlorination of cyclohexane. As shown in Supplementary Figs. 6 and 7 , the pristine TiO 2 photoanode exhibits a bandgap of 3.0 eV with an absorption wavelength of solar spectrum < 400 nm. This causes a relatively low photocurrent density of 1.5 mA cm −2 at 1.6 V vs. RHE in 0.5 M NaCl with 18.8 mmol cyclohexane under AM 1.5G illumination (100 mW cm −2 ). After introducing oxygen vacancy, the photocurrent density increases from 1.5 mA cm −2 (pristine TiO 2 ) to 3.4 mA cm −2 (TiO 2 -O v -400), suggesting the vital role of the oxygen vacancy for the PEC reaction activity. This can be partly attributed to the narrower bandgap of TiO 2 -O v -400 (2.75 eV; Fig. 3b and Supplementary Fig. 7 ) that facilitates photo-induced charge separation, suppresses electron-hole recombination, and also expands the light absorption range to visible light (from 410 nm to 450 nm). Noted that further increasing the H 2 treatment temperature (TiO 2 -O v -450) resulted in lower photocurrent density, which can be rationalized that the oxygen vacancy might induce photogenerated carriers recombination at higher concentration [30] . As a result, the TiO 2 -O v -400 exhibits better catalytic performance compared to other TiO 2 samples, achieving higher cyclohexane conversion rate, relatively higher selectivity (92.5%) and FE (77.5%) of chlorocyclohexane, and relatively lower FE of OER (7.3%) (Fig. 3b , Supplementary Fig. 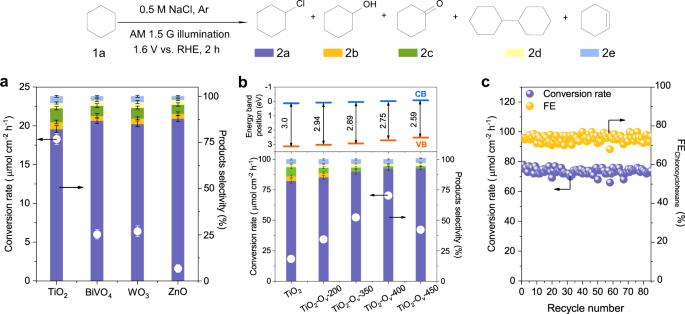Fig. 3: Cyclohexane chlorination performance via PEC. aPhotoelectrocatalytic conversion rate of cyclohexane and corresponding products selectivity over typical semiconductors.bPhotoelectrocatalytic conversion rate of cyclohexane and corresponding products selectivity over TiO2-Ov-T(Trepresents the temperatures, 200, 350, 400, and 450 °C) photoanodes.cStability test of TiO2-Ov-400 photoanode for the chlorination of cyclohexane for 255 h in batch reaction (85 batches). The reaction was carried out in a batch reaction in 0.5 M NaCl with 18.8 mmol cyclohexane at 1.6 V vs. RHE under AM 1.5G, 100 mW cm−2illumination, with 3 h for one batch. The spent TiO2-Ov-400 photoanode was washed by deionized water and dried under vacuum for the next batch reaction. The error bars represent the relative deviation, which is within 5%. The curves in each figure are guides to the eye. 8 and Supplementary Table 3 ). For the selectivity and FE calculations, all the organic products and evolved O 2 were included. The photon-to-current conversion efficiencies (IPCE) and photon-to-chlorocyclohexane quantum efficiency (QE) achieve 89.2% and 64.2% at a wavelength of 370 nm over TiO 2 -O v -400 (Supplementary Fig. 9 ), both higher than that of TiO 2 samples. The optimized PEC chlorination condition is presented as 0.5 M NaCl solution at 1.6 V vs. RHE under AM 1.5G illumination for 2 h (Supplementary Fig. 10 ), which was adopted for further catalytic reactions unless specified. The kinetic curves in Supplementary Fig. 11 show that chlorocyclohexane is the main product when the conversion of cyclohexane is lower than 60%. At this stage, cyclohexane underwent rapid oxidation, giving >50% yield of chlorocyclohexane with FE > 72%. However, chlorocyclohexane was partly converted to dichlorocyclohexane at higher cyclohexane conversion, and the conversion rate of cyclohexane gradually decreased, which is due to the involvement of highly reactive chlorine radicals that react with the accumulated chlorocyclohexane. Finally, we achieved a maximum chlorocyclohexane yield of 56.3% when the conversion of cyclohexane reached 63.1%. By using the PEC strategy, the organic halogenation reaction can be conducted in an energy-saving way by harnessing solar energy. To demonstrate it, we constructed an EC cell composed of a glass carbon anode, a Pt plate counter electrode and an Ag/AgCl reference electrode for the cyclohexane chlorination [12] (Supplementary Fig. 12 ). The results show that the applied bias to produce a (photo)-current of 2 mA cm −2 is 0.7 V vs. RHE for the TiO 2 -O v -400 PEC system, which is much lower than that of 2.4 V vs. RHE for the glassy carbon EC system. These potentials afford very similar cyclohexane conversion rates (41.2 µmol cm −2 h −1 in the PEC cell and 36.5 µmol cm −2 h −1 in the EC cell) and chlorocyclohexane selectivity (93% in the PEC cell and 90.7% in the EC cell) after 2 h of reaction, indicating the potential of energy-saving process for PEC organic synthesis. For the H 2 production performance at the counterpart Pt cathode, the space-time yield reaches 1.57 mL cm −2 h −1 over TiO 2 -O v -400, which is much higher than that of the pristine TiO 2 (0.66 mL cm −2 h −1 ; Supplementary Fig. 13 ). Both TiO 2 -O v -400 and pristine TiO 2 exhibit high Faradaic efficiency of H 2 (FE > 99%). We also evaluated the stability of the TiO 2 and TiO 2 -O v -400 photoanodes in PEC cyclohexane chlorination in batch reactions. As shown in Fig. 3c and Supplementary Fig. 14 , after 85 batches (overall 255 h), the conversion rate (from 70.0 to 69.2 µmol cm −2 h −1 ) and the FE of chlorocyclohexane (from 77.5 to 74.3%) remain stable, demonstrating the stability of the TiO 2 -O v -400 photoanode. Characterisations and photoelectric properties of the optimal TiO 2 -O v -400 The optimal TiO 2 -O v -400 photocatalyst was then characterised to understand the catalytic performance. X-ray diffraction (XRD) shows that TiO 2 -O v -400 displays a typical rutile phase of TiO 2 (Fig. 4a ) [32] . Scanning electron microscope (SEM) image reveals the formation of nanorod array structure with average diameter of 200–300 nm and length of ∼ 1.6 μm (Fig. 4b ). High-angle annular dark-field scanning transmission electron microscope (HAADF-STEM) images show that the nanorods are well crystallized with fringe distances of 0.323 nm and 0.289 nm (Fig. 4c ), closely matching the (110) and (001) plane of TiO 2 . The TiO 2 -O v -400 sample exhibits a strong electron paramagnetic resonance (EPR) signal at g value of 2.002 (Fig. 4d ), which can be attributed to the electrons trapped in oxygen vacancies [33] . Together with the XPS results shown above, these results further confirm the formation of oxygen vacancy in TiO 2 -O v -400. Fig. 4: Structural characterisations and photoelectric properties of TiO 2 -O v -400 photoanode. a XRD patterns of TiO 2 and TiO 2 -O v -400. b SEM images of TiO 2 -O v -400. Scale bars: 200 nm (inset). c HAADF-STEM images of the TiO 2 -O v -400. Scale bars: 200 nm, 2 nm (inset). d Room temperature EPR spectra of TiO 2 and TiO 2 -O v -400. e EPR spectrum detected from the photolysis of TiO 2 -O v -400 after immersing in 0.5 M NaCl under AM 1.5G (100 mW cm −2 ) illumination in toluene solution containing DMPO as spin-trapping agent. f Steady-state SPV spectra of TiO 2 and TiO 2 -O v -400 photoanodes. The inset shows the schematic of the photovoltaic cell structure. a.u. : arbitrary units. Full size image We then performed in-situ EPR and Cl 2 experiments to reveal the reaction mechanism of PEC chlorination of cyclohexane over TiO 2 -O v -400 photocatalyst. The EPR measurement was conducted in toluene by using 5,5-dimethyl-1-pyrroline N-oxide (DMPO) as the trapping agent [34] , [35] . As shown in Fig. 4e , both chlorine radical and carbon-centered radical were observed in the EPR spectrum after 5 min irradiation. After irradiation for 20 min, chlorine radical disappeared and carbon-centered radical remained in the system. This may be due to the quenching of chlorine radicals after it reacted with the C–H bond to yield carbon-centered radicals. Since chlorocyclohexane is the main product rather than C–C coupling products, the reaction mechanism should not follow a radical-radical combination process, but probably follow the free radical chain reaction. To further demonstrate the reaction mechanism, we used Cl 2 as the chlorine source for halogenation of cyclohexane. Cl 2 was injected into an aqueous solution containing 5 mmol cyclohexane in the presence of TiO 2 -O v or pure TiO 2 or without catalyst, and the reaction was performed under light irradiation or under darkness for 15 min. As shown in Supplementary Fig. 15a , under light irradiation, chlorocyclohexane is the only product for all the three reactions, and there are negligible products for reaction under darkness while other conditions were kept the same (Supplementary Fig. 15b ). Cl· was generated via the homolytic cleavage of Cl 2 under light irradiation, which follows a free-radical chain mechanism for cyclohexane chlorination [36] . As a result, the PEC halogenation of cyclohexane in our work probably follows a similar free-radical mechanism, except that Cl 2 was produced by direct oxidation of Cl − catalyzed by the photogenerated holes (h + ) over photoanode. To understand the high photoelectrocatalytic activity of the TiO 2 -O v -400 photoanode, its intrinsic photoelectric properties of TiO 2 -O v -400 were studied. Surface photovoltage (SPV) spectra provides a direct probe of the photophysics within semiconductor materials [37] . As shown in Fig. 4f , the TiO 2 -O v -400 exhibits an obvious steady-state SPV signal under light irradiation. The SPV signal decays with the increasement of excitation light wavelength, which corresponds to the excitation of oxygen vacancy. Clearly, introducing oxygen vacancy enhances the SPV response of TiO 2 , which demonstrates efficient photogenerated charge carrier separation efficiency. The photoluminescence (PL) emission spectra can be used to evaluate the recombination of photoexcited electrons/holes in TiO 2 , which shows the maximum broadbands around 470 nm [33] . As shown in Supplementary Fig. 16 , the TiO 2 -O v -400 sample exhibits lower intensity compared to the pristine TiO 2 and other TiO 2 -O v samples, demonstrating a more efficient separation of the photo-induced carriers. Moreover, the electrochemical impedance spectroscopy (EIS) plots present a faster kinetics of charge transfer at the interface of TiO 2 -O v -400 and the electrolyte (Supplementary Fig. 17 ), proving an efficient separation of the photo-induced carriers [38] . Effect of oxygen vacancy in promoting chloride ions oxidation We observed that TiO 2 -O v -400 shows higher photocurrent than pristine TiO 2 in a 0.5 M Na 2 SO 4 aqueous solution (dashed line, Fig. 5a ), indicating that TiO 2 with oxygen vacancy can also promote the activity of oxidation of H 2 O. However, the photocurrent increments for oxidation of Cl − is higher than oxidation of H 2 O. For the oxidation of Cl − at 1.6 V vs. RHE, the photocurrent was increased from 1.5 mA cm −2 (pristine TiO 2 ) to 3.4 mA cm −2 (TiO 2 -O v -400), that equals to 1.9 mA cm −2 enhancement. In contrast, for the oxidation of H 2 O at 1.6 V vs. RHE, the photocurrent was increased from 0.8 mA cm −2 (pristine TiO 2 ) to 1.9 mA cm −2 (TiO 2 -O v -400), showing 1.1 mA cm −2 enhancement. The inhibition of water oxidation of TiO 2 -O v -400 in 0.5 M NaCl was confirmed by online monitoring the O 2 generation rate and FE. As shown in Supplementary Fig. 18 , the FE of O 2 is <10% over TiO 2 -O v -400, lower than that over TiO 2 (~22%) under the conditions (in a 0.5 M NaCl solution after 1 h of reaction). These results indicate that the oxygen vacancy not only facilitates the photo-induced carriers separation efficiency over TiO 2 , but also has additional promoting effect for Cl − oxidation. Fig. 5: Mechanistic investigation of enriched Cl − at oxygen-vacancy sites. a LSV curves at scan rate of 10 mV s −1 in 0.5 M Na 2 SO 4 or NaCl electrolyte under AM 1.5G (100 mW cm −2 ) illumination. b Schematic diagram of the pretreatment process of TiO 2 -O v -400 and TiO 2 samples for further measurements (denoted as TiO 2 -O v -400-Cl and TiO 2 -Cl). c STEM combined EDS mapping images of TiO 2 -O v -400-Cl and TiO 2 -Cl. Scale bars: 100 nm. d Cl 2p XPS spectra of TiO 2 -O v -400-Cl and TiO 2 -Cl. e ARXPS spectra of Cl on TiO 2 -O v -400-Cl after Ar + sputtering. f IC spectrogram of NaCl solution after adsorbed by different TiO 2 -O v - T samples. g Cl − adsorption behavior of TiO 2 -O v -400 with different concentration of oxygen vacancy. h Adsorption energy of Cl − over TiO 2 and TiO 2 -O v . Inset: optimized geometries for TiO 2 and TiO 2 -O v adsorbed with Cl − , the color of each element is also labeled. a.u. : arbitrary units. Full size image We consider that it worth investigating the interaction between the TiO 2 with oxygen vacancy and Cl − . It is assumed that the Cl − upon adsorption would be difficult to remove by moderate washing treatment and retain on the TiO 2 surface if a strong interaction exists between them, then the remained Cl − can be detected. For this consideration, as illustrated in Fig. 5b , TiO 2 -O v -400 and pristine TiO 2 were firstly immersed in a 0.5 M NaCl solution under continuous stirring for 1 h to fully adsorb Cl − . Then, they were washed by deionized water and dried under vacuum (denoted as TiO 2 -O v -400-Cl and TiO 2 -Cl, respectively) for further analysis. The energy-dispersive X-ray spectroscopy (EDS) mapping results in Fig. 5c and Supplementary Fig. 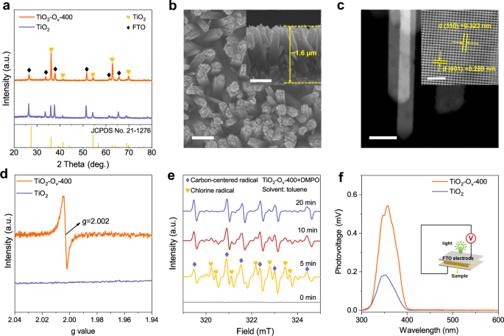Fig. 4: Structural characterisations and photoelectric properties of TiO2-Ov-400 photoanode. aXRD patterns of TiO2and TiO2-Ov-400.bSEM images of TiO2-Ov-400. Scale bars: 200 nm (inset).cHAADF-STEM images of the TiO2-Ov-400. Scale bars: 200 nm, 2 nm (inset).dRoom temperature EPR spectra of TiO2and TiO2-Ov-400.eEPR spectrum detected from the photolysis of TiO2-Ov-400 after immersing in 0.5 M NaCl under AM 1.5G (100 mW cm−2) illumination in toluene solution containing DMPO as spin-trapping agent.fSteady-state SPV spectra of TiO2and TiO2-Ov-400 photoanodes. The inset shows the schematic of the photovoltaic cell structure. a.u.: arbitrary units. 19 reveal that Cl species are uniformly distributed on the surface of the TiO 2 -O v -400-Cl with mass loading of ~0.67 wt% (Supplementary Table 4 ). In contrast, there is no obvious Cl on the surface of the TiO 2 -Cl. XPS measurement (Fig. 5d ) show that TiO 2 -O v -400-Cl exhibits a set of typical Cl 2p XPS peaks at 198.1 eV (Cl 2p 3/2 ) and at 199.8 eV (Cl 2p 1/2 ) [39] , while they are absent in the TiO 2 -Cl sample. These results suggest that TiO 2 -O v -400 adsorbs Cl − stronger than the pristine TiO 2 that is due to the oxygen vacancy. To investigate the location of the adsorbed Cl over the TiO 2 -O v -400-Cl, namely on the surface or in the bulk, angle-resolved XPS (ARXPS) was conducted. The results show that the peak intensities of Cl 2p on the TiO 2 -O v -400 became less intensive and finally disappeared with the extension of Ar + sputtering time (from 0 to 200 s; Fig. 5e ), indicating that Cl − is mainly adsorbed on the surface of TiO 2 -O v -400. We then estimated the adsorption quantity of Cl − by immersing TiO 2 -O v - T samples in a NaCl aqueous solution and then measuring the Cl − concentration in the NaCl solution using ion chromatography (IC; Fig. 5f , Supplementary Fig. 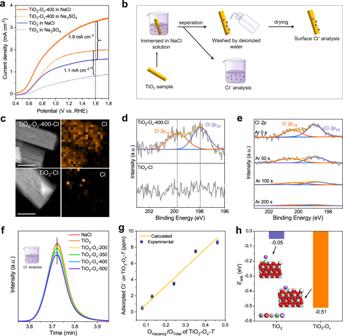Fig. 5: Mechanistic investigation of enriched Cl−at oxygen-vacancy sites. aLSV curves at scan rate of 10 mV s−1in 0.5 M Na2SO4or NaCl electrolyte under AM 1.5G (100 mW cm−2) illumination.bSchematic diagram of the pretreatment process of TiO2-Ov-400 and TiO2samples for further measurements (denoted as TiO2-Ov-400-Cl and TiO2-Cl).cSTEM combined EDS mapping images of TiO2-Ov-400-Cl and TiO2-Cl. Scale bars: 100 nm.dCl2pXPS spectra of TiO2-Ov-400-Cl and TiO2-Cl.eARXPS spectra of Cl on TiO2-Ov-400-Cl after Ar+sputtering.fIC spectrogram of NaCl solution after adsorbed by different TiO2-Ov-Tsamples.gCl−adsorption behavior of TiO2-Ov-400 with different concentration of oxygen vacancy.hAdsorption energy of Cl−over TiO2and TiO2-Ov. Inset: optimized geometries for TiO2and TiO2-Ovadsorbed with Cl−, the color of each element is also labeled. a.u.: arbitrary units. 20 and Supplementary Table 5 ). Based on the measurement results, the adsorbed amount of Cl − has a positive correlation with the concentration of oxygen vacancy on TiO 2 -O v - T (Fig. 5g ), demonstrating that the oxygen vacancy on TiO 2 has a pivotal role in Cl − adsorption and may enrich Cl − in local environment on TiO 2 surface for enhanced catalytic performance. Spin-polarized density functional theory studies Spin-polarized density functional theory (DFT) calculations were performed to reveal the effect of oxygen vacancy on the adsorption of Cl – , and its further oxidation to Cl· and Cl 2 on TiO 2 -O v , together with the chlorination of cyclohexane by Cl· and Cl 2 in solvent. Detailed information for model construction and computational methods are presented in the Methods section. According to the HAADF-STEM results (Fig. 4c ), the exposed facet of TiO 2 -O V is determined to be the (101) facet, which has been reported to be one of the preferably exposed facets of rutile TiO 2 [40] . By calculating the Gibbs free energies of TiO 2 (101) facets terminated with Ti, –H, –OH, and –O species, it is found that the (101) facet terminated with –OH is more stable than the others (Supplementary Figs. 21 and 22 , and Supplementary Note 1 ). Therefore, the TiO 2 (101) facet terminated with –OH was employed in the following calculations. As shown in Fig. 5h , the Cl ‒ is adsorbed on the oxygen vacancy of TiO 2 -O v with a moderate adsorption energy of –0.51 eV, resulting from the orbital overlap between the occupied Cl-3 p orbital in Cl ‒ and unoccupied Ti-3 d orbital. In contrast, the adsorption of Cl ‒ on TiO 2 is much weaker than that on TiO 2 -O v because of the repulsion between the lone pair electrons of Cl ‒ and that of bridged O in TiO 2 , resulting in the adsorption energy of –0.05 eV (Fig. 5h and Supplementary Fig. 23 ). These theoretical results well explain the moderate adsorption of Cl ‒ on TiO 2 -O v -400 photoanode according to the experimental results (Fig. 5c–g ). According to the Sabatier rule [41] , too weak adsorption of reactant may lead to a slow reaction rate, as in the case with TiO 2 . While TiO 2 -O v possesses an intermediary adsorption strength to Cl – , facilitating the adsorption of Cl – , generation and desorption of Cl*. Furthermore, the Gibbs free energy diagrams of the whole process for the chlorination of cyclohexane over TiO 2 -O v were calculated. As shown in Fig. 6a , after the adsorption of Cl – on TiO 2 -O v , the Cl – is oxidized by the hole of TiO 2 -O v spontaneously with a Gibbs free energy change (Δ G ) of –1.28 eV. The potential determining step is the desorption of Cl* to Cl· with a Δ G of 0.78 eV, which can be overcome by the kinetic energy of Cl* at room temperature. After the recovery of the active site, another Cl – is adsorbed on the oxygen vacancy, which is followed by the oxidation of Cl – to Cl*. After that, another Cl – is oxidized by the hole on Cl*, generating Cl 2 * exothermically with a Δ G of –2.73 eV. Then the Cl 2 desorbs spontaneously from the oxygen vacancy of TiO 2 -O v with a Δ G of –0.08 eV. Noted that Cl 2 may be also formed by dimerization of two Cl· that desorbed from the surface of TiO 2 -O v . After that, the generated Cl· and Cl 2 chlorinate the cyclohexane in solvent. Firstly, the Cl· reacts with the C‒H bond in cyclohexane to generate carbon-centered radical exothermically with a Δ G of –0.20 eV. Then, the generated carbon-centered radical reacts with the Cl 2 to give chlorocyclohexane and release the Cl· for the next cycle spontaneously with a Δ G of –0.91 eV. The proposed mechanism of PEC cyclohexane chlorination is presented in Fig. 6b : i. chlorine radicals (Cl·) are generated through the activation of Cl – by the photogenerated holes (h + ) over TiO 2 -O v -400 or TiO 2 photoanode via single electron transfer; ii. the generated Cl· then activates the C–H bonds of cyclohexane to form cyclohexane radical. Cl 2 can be generated by dimerization of two Cl· or by oxidation of two Cl − catalyzed by the photogenerated holes (h + ) over TiO 2 ; iii. the generated cyclohexane radical reacts with Cl 2 to form chlorocyclohexane and release the Cl· for the next cycle. The chlorocyclohexane can be further chlorinated to form dichlorocyclohexane following the same free-radical mechanism. Fig. 6: DFT calculations of the PEC cyclohexane chlorination and proposed mechanism. a Gibbs free energy diagram for the adsorption of Cl – , generation of Cl* and Cl 2 *, and their further desorption to Cl· and Cl 2 on TiO 2 -O v , together with the chlorination of cyclohexane by Cl· and Cl 2 . The Gibbs free energies (Δ G ) of reactant, intermediates, and product are labeled with blue numbers in brackets with the unit of eV. The Δ G of the potential determining step, desorption of Cl*, is labeled in red number with the unit of eV. The top views for the reaction intermediates, * (the reaction site of oxygen vacancy is highlighted with green circle), Cl – *, Cl*, and Cl 2 *, are also displayed with the color of each element labeled. b Proposed mechanism of PEC chlorination of cyclohexane over TiO 2 -O v -400 photoanode. Full size image Scope of photoelectrocatalytic C–H halogenation To demonstrate the general applicability of the photoelectrocatalytic strategy for C–H halogenation over the TiO 2 -O v -400 photoanode, a broad scope of substrates was tested, including arenes, heteroarenes, nonpolar cycloalkanes, and aliphatic hydrocarbons. As shown in Table 1 , for aromatic compounds with strong electron-donating groups (e.g., anisole and phenol; 1 and 2), di-chlorinated products were mainly obtained under high conversion (>90%), with selectivity of 52.6% for 2,4-dichloro-1-methoxybenzene (1) and 51.5% for 2,4-dichlorophenol (2) (Supplementary Figs. 24 and 25 ). For aromatic compounds with strong electron-withdrawing halogen groups (3–5), mono-chlorinated products were mostly obtained with the regioselectivities (the ratio of para - to ortho- , p / o ) approximately of 1:0.7 to 1:1 (Supplementary Figs. 26 , 27 , and 28 ). It should be noted that for aromatic compounds with methyl group (e.g., toluene and methylnaphthalene; 6 and 7), aromatic ring-chlorinated compounds were the major products rather than the methyl-chlorinated ones (Supplementary Figs. 29 and 30 ). This is due to the PEC chlorination of toluene and methylnaphthalene over TiO 2 -O v -400 photoanode mainly follows an electrophilic substitution mechanism, which was demonstrated by the chlorine gas (Cl 2 ) experiment (Supplementary Figs. 31 – 33 ; please see the detailed discussion in Supplementary Note 2 in the Supplementary information ). For aromatic substrate with singular reactive site (vanillin, 8), high 5-chlorovanillin selectivity (>99%) were achieved under high conversion (94.2%) (Supplementary Fig. 34 ). Moreover, the TiO 2 -O v -400 photoanode can realize the PEC chlorination of heteroarenes (including thiophene, pyrazole, indoles, pyridine, furan, and imidazole-based substrates; 9–15), affording mono- or di-chlorinated products under high conversion (Supplementary Figs. 35 – 41 ). We then attempted to extend the substrate to drug-related compound, anesthetic procaine (16), and high selectivity of chloroprocaine was obtained, although the conversion (23.2%) was not improved significantly as the reaction time were prolonged, which is attributed to the steric hindrance of the benzene ring with large function group (Supplementary Fig. 42 ). Table 1 Scope of PEC C−H halogenation over TiO 2 -O v -400 photoanode. Full size table For nonpolar cycloalkanes (17–19), mono-chlorinated products were the main products under high conversion (Supplementary Figs. 43 – 45 ). The chlorination of cycloalkanes with chlorine group (20 and 21) and methyl group (22) took place in the tertiary C − H bond position (Supplementary Figs. 46 – 48 ) because it is more reactive. To our delight, the PEC strategy is applicable to chlorination of alkanes including n -pentane and n -hexane (23, 24), and the chlorination mostly occurred in the tertiary C−H bond position (Supplementary Figs. 49 and 50 ). Because n -pentane and n -octane are highly volatile, some technical challenge remains to achieve high conversion by using the unsealed PEC reactor in our work. We are working on developing airtight reactor to overcome this challenge. Most of the products are detectable on GC, as evidenced by the comparable yield and conversion data that suggests the polymerization and other side reactions can be largely neglectable. Moreover, the halide anion used in the PEC halogenation can be extended from Cl − to Br − , and I − using NaBr and NaI as the reactants, respectively, achieving bromination and iodination reactions have been achieved (25–27; Supplementary Figs. 51 – 53 ), demonstrating the generality of the PEC halogenation strategy. PEC halogenation based on seawater For a practical application, we sought to perform the halogenating reaction coupled with H 2 production by directly using seawater as both the electrolyte and Cl − source, which provides a route to directly use renewable solar and ocean resource for recycling of halogen into valuable chemicals. Natural seawater used in this work was collected from the Yellow Sea (36.0532°N, 120.4115°E), Shandong Province, China, with chloride ion concentration of ∼ 18 g L −1 (determined by ion chromatography; Fig. 7a ). The pH of the natural seawater was measured to be 7.4 after simply filtering out silts and algae microorganisms, etc. We then evaluated the PEC halogenation performance of TiO 2 -O v -400 in the natural seawater with 0.5 M of cyclohexane in H-type quartz cell. As shown in Fig. 7b , the TiO 2 -O v -400 exhibits an obviously enhanced photocurrent under AM 1.5G (100 mW cm −2 ) illumination. Specifically, the photocurrent density reaches 4.6 mA cm −2 at 1.6 V vs. RHE with chlorocyclohexane production rate of 64.5 μmol cm −2 h −1 and selectivity of 88.6% (Fig. 7c and Supplementary Fig. 54a ). The production rate of chlorocyclohexane could be further improved with the increase of potential, but the production rate of the by-products would also increase (Fig. 7c and Supplementary Fig. 54b ). The long-term stability of TiO 2 -O v -400 photoanode in seawater was also examined. As shown in Fig. 7d , the photocurrent density of TiO 2 -O v -400 maintained ~98% after 150 h at 1.6 V vs. RHE under AM 1.5G (100 mW cm −2 ) illumination in seawater. Moreover, the initial nanoarray structure and the oxygen-vacancy are stable for TiO 2 -O v -400 photoanode (Supplementary Fig. 55 ). The vacancy-related properties of TiO 2 -O v -400 photoanode were largely maintained, such as the light absorption range, energy band position (2.75 eV), the photo-induced charge separation efficiency and the charge transfer properties (Supplementary Fig. 56 ), demonstrating the high stability of TiO 2 -O v -400 photoanode. Fig. 7: PEC chlorination based on seawater. a The concentration of the main anions in the natural seawater collected from the Yellow Sea, Shandong Province, China. b LSV curves at scan rate of 10 mV s −1 of TiO 2 -O v -400 photoanode in seawater under AM 1.5G (100 mW cm −2 ) illumination (solid line) or in the dark (dashed line). c Production rate of chlorocyclohexane on TiO 2 -O v -400 photoanode using seawater as electrolyte under AM 1.5G (100 mW cm −2 ) illumination at different potentials for 2 h in an H-type photoelectrocell. d Current-time ( I-t ) curve of TiO 2 -O v -400 for PEC cyclohexane chlorination in seawater for 150 h reaction. e Schematic illustration of the self-powered PEC system. f The photo of the self-powered PEC system under AM 1.5G (100 mW cm −2 ) illumination. g Productivity of the PEC chlorination products in self-powered PEC system. The error bars represent the relative deviation, which is within 5%. Full size image In addition, we designed a self-powered PEC system, which is equipped with a solar panel (~2 V) to provide constant bias, a homemade PEC flow cell with TiO 2 -O v -400 photoanode, and seawater was directly utilised as the electrolyte and Cl − source (Fig. 7e, f ). As shown in Fig. 7g , this self-powered PEC system successfully achieved C–H halogenation of cyclohexane with chlorocyclohexane productivity of 3.3 mmol (~412 µmol h −1 ) and H 2 productivity of ~9.2 mL h −1 after 8 h of reaction under AM 1.5G illumination (100 mW cm −2 ), demonstrating the potential of the PEC strategy in using seawater for sustainable organic halides production. In summary, we achieved a highly efficient PEC C–H halogenation in a neutral aqueous solution to produce high value-added organic halides and promote cathodic H 2 production by using an oxygen-vacancy-rich TiO 2 photoanode. Experimental studies and DFT calculations reveal that the halide ions can be adsorbed at the oxygen-vacancy sites of photoanode, which promotes the oxidation of halide ions to free-radical and followed C–H halogenation process. We confirm that this PEC strategy exhibits broad substrate scope including arenes, heteroarenes, nonpolar cycloalkanes, and aliphatic hydrocarbons. Moreover, we designed a self-powered PEC system and directly utilized seawater as the electrolyte and the Cl − source, which achieved chlorocyclohexane productivity of 412 µmol h −1 coupled with H 2 productivity of 9.2 mL h −1 . This work may open a promising sustainable approach for photoelectrochemical C–H halogenation coupling H 2 production under mild conditions. It should be noted that while the electrocatalysis (especially photovoltaics combined with electrolysis system) shows higher energy conversion efficiency in many catalytic reactions than PEC does, it is still important to develop PEC technology because it is ideally powered by sunlight [2] . PEC technology is still in its infancy and many fundamental and technical challenges remain that make it currently less competitive with electrocatalysis, such as the low energy efficiency and relatively lower catalyst activity. Nevertheless, the continuous innovation of the advanced photoelectrocatalysts and PEC devices with enhanced efficiency [31] have shed light on PEC application in the future. We believe that the synergetic development of electrocatalysis, photocatalysis, and PEC technologies for material synthesis and energy conversion is essential to establish a sustainable society that doesn’t rely on fossil fuels. General information Except noted, all chemicals were purchased and used without further purification. Catalyst preparation Preparation of TiO 2 photoanode TiO 2 nanorod array was prepared via a facile hydrothermal method [32] . Initially, the fluorine doped conductive SnO 2 (FTO, 7 Ω, light transmittance 80%, active area 20 × 20 × 2.2 mm) was sequentially washed with solution containing acetone, isopropanol, and deionized water (1:1:1) to remove surficial contaminants. Then, 0.175 mL of titanium butoxide was dropwise added into a H 2 O/HCl mix solution with equal volume (6 mL) of H 2 O and HCl (36.5–38 wt%) under continuous stirring. The resulting solution and the pre-treated FTO substrate were transferred and sealed in a Teflon-lined stainless-steel autoclave (25 mL) and heated to 150 °C for 20 h. The as-obtained TiO 2 nanorod array was removed from the autoclave, washed thoroughly with distilled water and dried in air, then followed by annealing at 350 °C in an ambient environment for 2 h (heating rate: 5 °C min −1 ) to improve the crystallinity of TiO 2 nanorods and enhance their contact to the FTO substrate. Preparation of TiO 2 -O v photoanode The pristine TiO 2 nanorod array was annealed in H 2 atmosphere (10% H 2 and 90% Ar) at various temperatures (200, 350, 400, and 450 °C) for 2 h (heating rate: 5° min −1 ). The H 2 -treated samples are denoted as TiO 2 -O v - T ( T represents the temperatures, 200, 350, 400, and 450 °C). Preparation of WO 3 photoanode WO 3 nanosquare array was prepared via a facile hydrothermal method [42] . Typically, 6 mL of HCl (3 M) was dropwise added into Na 2 WO 4 ·2H 2 O (10 mM) solution under constant stirring at room temperature. Subsequently, 0.2 g of (NH 4 ) 2 C 2 O 4 was added into the above suspension and deionized water was added to 70 mL with continual stirring for 30 min. The resulting solution and the pre-treated FTO substrate were transferred and sealed in a Teflon-lined stainless-steel autoclave (25 mL) and heated to 150 °C for 2 h. The as-obtained WO 3 precursor simple was washed thoroughly with distilled water and calcined in air at 450 °C for 2 h (heating rate: 5 °C min −1 ) to obtain WO 3 nanosquare array photoanode. Preparation of BiVO 4 photoanode BiVO 4 photoanode was synthesised following a two-step method [43] . Firstly, Bi-metal was electrodeposited onto the FTO substrate (Bi@FTO). The room temperature electrodeposition was carried out in a three-electrode configuration using an electrochemical workstation (CHI 760E, CH Instrument Co. USA), and was accomplished by holding the FTO electrode at −0.6 V (vs. Ag/AgCl) for 600 s while the FTO was in contact with an aqueous solution of 1 mmol Bi(NO 3 ) 3 ·5H 2 O in 50 mL of water and 100 mL ethylene glycol. The electrodeposited Bi was then washed with ethanol. The as-obtained the Bi@FTO samples were dipped in 0.2 mL VO(acac) 2 dimethyl sulfoxide (DMSO) solution (0.2 M). The samples were then heated in air at 450 °C for 2 h (heating rate: 2 °C min −1 ). The samples were then left to cool naturally to ambient temperature. Residual V 2 O 5 was removed by stirring the samples in 1 M NaOH. Finally, the BiVO 4 photoanode was cleaned by deionized water and dried in air. Preparation of ZnO photoanode ZnO nanowire array were prepared by a facile hydrothermal method [44] . Briefly, 100 mL of a 0.1 M solution of Zn(CH 3 COOH) 2 in absolute ethanol was prepared with ultrasonic agitation. A thin layer of ZnO seeds were obtained by spin-coating of the above solution on the FTO substrates, followed by annealing at 350 °C for 30 min. The seeded substrates were sealed in a reagent solution containing 0.1 M Zn(NO 3 ) 2 and 0.1 M HMT in an autoclave and then heated to 110 °C for 24 h for nanowire growth. The nanowire substrate was removed from the autoclave, washed thoroughly with distilled water and dried in air. Sample characterizations X-ray powder diffraction (XRD) patterns were recorded using a Shimadzu XRD-6000 diffractometer equipped with a graphite-filtered Cu Kα radiation source ( λ = 0.15418 nm). X-ray photoelectron spectra (XPS) were performed on a Thermo VG ESCALAB 250 X-ray photoelectron spectrometer at a pressure of about 2 × 10 −9 Pa using Al Kα X-rays as the excitation source. Scanning electrode microscope (SEM) images were taken on a Zeiss SUPRA 55 Field Emission scanning electron microscope operated at 20 kV. Transmission electron microscopy (TEM) images were recorded with JEOL JEM-2010 high resolution (HR-)TEM operated at 200 kV, combined with energy dispersive X-ray spectroscopy (EDX). Powder samples used in this work were scraped from the TiO 2 nanoarray-FTO glass. UV–vis diffuse reflectance spectrum was recorded in the spectral region of 300–800 nm on a Shimadzu UV-3000 spectrophotometer. Photoluminescence (PL) spectra were obtained at ambient temperature using a HitachiF-7000 fluorescence spectrophotometer with an excitation wavelength of 300 nm. The bandgap of samples was determined based on the Tauc plot. The steady-state and transient surface photovoltage (SPV) measurements were performed on a lock-in amplifier (SR830-DSP) with a light chopper (SR540) and a photovoltaic cell. A 300 W xenon lamp in conjunction with a double-prism monochromator (Zolix SBP500) provided monochromatic light as the light source. The concentration of chloride ion in solution was analyzed using the ion chromatography (IC, 2016 Timebase ICS-5000). Room-temperature EPR spectra of samples were collected on a JES-FA200 X ESR spectrometer (298 K, 9063.386 MHz). 5,5-Dimethyl-1-pyrroline N-oxide (DMPO) was used as the spin-trapping agent. 0.5 mg samples were dispersed in 2 mL toluene, then 50 µL DMPO was added into the solution, and after filled with argon irradiated with 300 W Xenon lamp (Microsolar 300; Beijing Perfectlight) with an AM 1.5G filter (100 mW cm −2 ) for ESR measurement. Photoelectrochemical characterization Photoelectrochemical measurements were conducted on an electrochemical workstation (CHI 760E, CH Instruments, Inc.) using a sealed H-type glass cell in a three-electrode system (Ag/AgCl electrode as reference electrode and Pt foil as counter electrode). Nafion proton exchange membrane was used to separate the photoanode from the cathode chamber. The simulated solar illumination was obtained from a 300 W Xenon lamp with an AM 1.5 G filter (100 mW cm −2 ). The electrolyte contains 0.5 M NaCl aqueous solution. Photocurrent was recorded from 0.4 to 1.8 V vs. RHE at a scan rate of 10 mV s −1 with the presence of cyclohexane. All potentials mentioned in this work were converted to potentials versus RHE (in volts) according to Eq. 1 : 
    E_RHE=E_Ag/AgCl+E_Ag/AgClvs.NHE+0.059pH
 (1) Where E Ag/AgCl vs. NHE in Eq. 1 is 0.197 V at 20 °C. The photoelectrochemical impedance spectra were collected in a frequency range of 1~10 5 Hz with an amplitude of 1 mV under AM 1.5G, 100 mW cm −2 illumination, from 0.4 V to 1.8 V vs. RHE. Mott–Schottky plots were measured at 1500 Hz in dark with potential varied from −0.4 to 1.0 V vs. RHE. IPCE was measured under monochromatic irradiation under one sun illumination (AM 1.5 G, 100 mW cm −2 ) equipped with a monochromator at 1.6 V vs. RHE: 
    IPCE= [(1240/λ)× (J_light-J_dark)]/P× 100 %
 (2) where λ is the wavelength, J light is the photocurrent density under irradiation, J dark is the current density under dark condition, and P is the incident light power density. Photoelectrocatalysis characterizations Under general reaction conditions, the photoanode was immersed in 0.5 M NaCl (20 ml) containing cyclohexane (2 mL, 18.8 mmol) in a sealed H-type cell, and Ar was bubbled through the solution for 30 min. The solution was stirred continuously at 500 rotations min −1 . Then, the photoelectrochemical chlorination was performed at a potential of 1.6 V vs. RHE for 2 h under AM 1.5G, 100 mW cm −2 illumination, and the temperature was maintained at room temperature (around 298 K). After reaction, 1 mL of solution was taken out from the cell and analyzed using gas chromatography mass spectrometry (GC-MS, Agilent Technologies, GC7890B, MS 5977B) to identify production or dissolve in 2 mL absolute ethanol for further quantitative analysis using an Agilent chromatograph equipped with a HP-5 (300 × d mm, 8 μm) column and FID detector. Selectivity of products was calculated based on: 
    Selectivity= content of corresponding product detected via GC/consumption of reactant× 100 %
 (3) 
    Conversion rate=consumption of reactant/t× A
 (4) where t is the reaction time (h), and A is the area of photoanode (cm −2 ). Faradaic efficiency was calculated by: 
    Faradaic efficiency=e_products×n_products× N/Q/n× 100 %
 (5) where e products is the number of holes required to oxidize cyclohexane/H 2 O molecule to products, including chlorocyclohexane ( e = 2), cyclohexanol ( e = 2), cyclohexene ( e = 2), bicyclohexyl ( e = 2), cyclohexanone ( e = 4), O 2 ( e = 4). n products is the productivity of products, N is Avogadro’s constant ( N = 6.02 × 10 23 ), Q is the quantity of electric charge, and n is the elementary charge ( e = 1.602 × 10 −19 C). The external quantum efficiency of photon-to-products was calculated based on IPCE and faradaic efficiency of products. External quantum efficiency of DHA was calculated by: 
    QE 	= Number of holes to chloridize cyclohexane /Number of incident photons× 100 %
     	= IPCE×Faradaic efficiency× 100 %
 (6) Oxygen production was measured using a Neo-FOX oxygen-sensing system (Ocean Optics Inc.) equipped with a FOX Y probe inserted into the headspace of an airtight cell. The cell was purged with nitrogen for 2 h prior to measurement. The oxygen fluorescence signal was allowed to stabilize after the nitrogen flow was stopped. Once the residual oxygen signal was constant, bias was applied to the electrode. 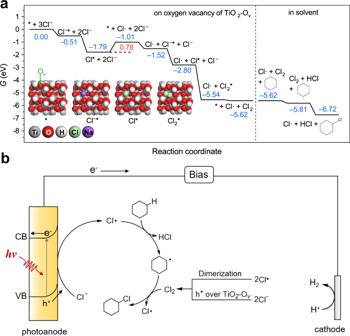Fig. 6: DFT calculations of the PEC cyclohexane chlorination and proposed mechanism. aGibbs free energy diagram for the adsorption of Cl–, generation of Cl* and Cl2*, and their further desorption to Cl· and Cl2on TiO2-Ov, together with the chlorination of cyclohexane by Cl· and Cl2. The Gibbs free energies (ΔG) of reactant, intermediates, and product are labeled with blue numbers in brackets with the unit of eV. The ΔGof the potential determining step, desorption of Cl*, is labeled in red number with the unit of eV. The top views for the reaction intermediates, * (the reaction site of oxygen vacancy is highlighted with green circle), Cl–*, Cl*, and Cl2*, are also displayed with the color of each element labeled.bProposed mechanism of PEC chlorination of cyclohexane over TiO2-Ov-400 photoanode. 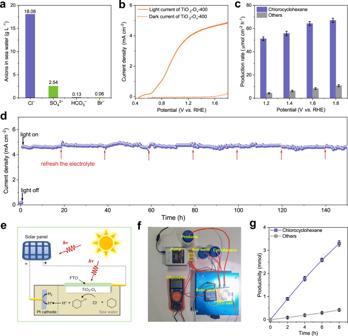Fig. 7: PEC chlorination based on seawater. aThe concentration of the main anions in the natural seawater collected from the Yellow Sea, Shandong Province, China.bLSV curves at scan rate of 10 mV s−1of TiO2-Ov-400 photoanode in seawater under AM 1.5G (100 mW cm−2) illumination (solid line) or in the dark (dashed line).cProduction rate of chlorocyclohexane on TiO2-Ov-400 photoanode using seawater as electrolyte under AM 1.5G (100 mW cm−2) illumination at different potentials for 2 h in an H-type photoelectrocell.dCurrent-time (I-t) curve of TiO2-Ov-400 for PEC cyclohexane chlorination in seawater for 150 h reaction.eSchematic illustration of the self-powered PEC system.fThe photo of the self-powered PEC system under AM 1.5G (100 mW cm−2) illumination.gProductivity of the PEC chlorination products in self-powered PEC system. The error bars represent the relative deviation, which is within 5%. The oxygen evolution was monitored at 1.6 V vs. RHE. The space-time yield of H 2 was obtained by gas-collecting method of drainage water. For long-term photoelectrochemical measurement by constant potential (CP) strategies, the productivity of H 2 was calculated based on the charge transfer of cyclohexane chlorination. Computational details Model construction Two models named as TiO 2 -O v and TiO 2 were constructed to represent the photoanode TiO 2 -O V -400 used in this work and the control sample TiO 2 without oxygen vacancy, respectively. Firstly, the model of bulk rutile TiO 2 was constructed according to the single crystal X-ray diffraction measurement in previous literature [45] . The space group of rutile TiO 2 is P42/mnm, with the lattice parameters of a = b = 4.59 Å, c = 2.96 Å, α = β = γ = 90°. According to the HAADF-STEM image of TiO 2 -O v -400 (Fig. 2c ) that displays the interplanar spacings of (110) and (101) facets, the exposed facet of TiO 2 -O v -400 is deduced to be the (011) facet, which is perpendicular to the (110) and (101) facets. Since rutile TiO 2 is isotropic in the lattice a and b directions, the (011) facet is identical to the (101) facet. Moreover, the (101) facet has been widely reported to be one of the preferably exposed facets of rutile TiO 2 [38] . Thus the (101) facet of rutile TiO 2 was cleaved, containing four layers of Ti atoms, eight layers of O atoms, and a vacuum layer of 20 Å. According to the previous literature, the surface of TiO 2 may be passivated by OH* or H* (* represents the surface of rutile TiO 2 ) in aqueous environment [46] , [47] , [48] , [49] , therefore, under the reaction condition here (1.6 V vs. RHE), the surface of TiO 2 -O V may be covered with ‒H, –OH, or –O, or terminated with Ti. Thus, four surface models terminated with Ti, –H, –OH, and –O were constructed and named as S1, S2, S3, and S4, respectively (Supplementary Note 2 ). The optimized geometries of models S1, S2, S3, and S4 are displayed in Supplementary Fig. S24 . Then the Gibbs free energies of these four facets were calculated referred to the method proposed by Valdes et al [50] and displayed in Supplementary Fig. S25 . It was found that the surface S3 where the coordination unsaturated Ti atoms are covered by the OH* are the most stable with the lowest Gibbs free energy among S1, S2, S3, and S4 under reaction condition, 1.6 V vs. RHE (Supplementary Fig. S25 ). Therefore, the facet S3 with the chemical formula of Ti 32 O 77 H 8 is used as model TiO 2 -O V in the following calculations. The chemical formula of model TiO 2 is Ti 32 O 80 H 8 . The amount of oxygen vacancy on model TiO 2 -O v is 37.5% on the surface, which was referred to the X-ray photoelectron spectra result that the amount of oxygen vacancy is 35% on the surface of TiO 2 -O v -400 (Supplementary Table 2 ). When calculating the mechanism of the generation of Cl* and Cl 2 * on TiO 2 -O v , the intermediate models of Cl – * (one Na + cation was added to keep the model neutral), Cl*, and Cl 2 * were constructed. For each intermediate model, the possible adsorption sites of top, bridge, and fcc sites were screened to find the optimal adsorption site. Computational methods Spin-polarized DFT calculations were performed with the plane wave implementation in Cambridge Sequential Total Energy Package (CASTEP) [51] . The Perdew-Burke-Ernzerhof (PBE) in generalized gradient approximation (GGA) was used as the exchange-correlation functional [52] . The ionic core of Ti was described with the ultrasoft pseudopotentials to improve transferability and reduce the number of plane waves needed to expand the Kohn-Sham orbitals. The cutoff energy was set as 400 eV and the k -point meshes was set as 3 × 3 × 1 [53] . To validate the convergence of the basis set size, the Δ G for the desorption of Cl* was calculated with a 600 eV cut-off. The Δ G varied by less than 0.015 eV, supporting the choice of 400 eV cutoff in this work. To validate the convergence of k -point meshes, the Δ G for the desorption of Cl* was calculated with a 5 × 5 × 1 k -point meshes. The Δ G varied by less than 0.010 eV, indicating that the 3 × 3 × 1 k -point meshes was converged. The Broyden-Fletcher-Goldfarb-Shanno (BFGS) algorithm was used to search the potential energy surface during geometry optimization [54] . The following three points were used during geometry optimization: (1) a maximum energy tolerance of 1.0 × 10 –6 eV per atom, (2) a maximum force tolerance of 3.0 × 10 –2 eV/Å, and (3) a maximum displacement tolerance of 1.0 × 10 –3 Å. Proposed mechanism It is proposed that the chlorination of cyclohexane mainly follows a free-radical reaction mechanism [20] , [36] . Since chlorocyclohexane is the main product rather than C–C coupling products for photoelectrochemical chlorination of cyclohexane in this work, the chlorination of cyclohexane probably follows the free-radical chain reaction mechanism. The reaction formula of the chlorination of cyclohexane in this work is deduced to be as follows: 
    ∗ +Cl^-→Cl^-∗ (∗represents the reaction site)
 (A) 
    Cl^-∗→Cl∗ +e^-
 (B) 
    Cl^∗ → ^∗+Cl·
 (C) 
    ∗ +Cl^-→Cl^-∗
 (D) 
    Cl^-∗→Cl∗ +e^-
 (E) 
    Cl^∗+Cl^-→Cl_2^∗+e^-
 (F) 
    Cl -2.2pt· + Cl·→Cl_2(in solvent)
 (G) 
    Cl_2^∗ → ^∗+Cl_2
 (H) 
    Cl· + C_6H_12→C_6H_11· + HCl
 (I) 
    Cl_2+C_6H_11·→C_6H_11Cl+HCl
 (J) The Δ G of each elementary step was obtained by minus the Gibbs free energy of reactant with that of product. The Gibbs free energy of (Na + + e – ) was treated with the standard electrode potential of Na + /Na (–2.714 V vs. RHE) [55] referred to the computational standard hydrogen electrode approximation [51] . The driving force of photo-induced hole on TiO 2 -O v is determined to be 2.6 eV according to its band edge placement of valence band maximum (2.6 V vs. NHE, Supplementary Fig. 7d ). The influence of bias was treated with the computational standard electrode potential approximation C6 with the term “– eU ”. The Gibbs free energy of reactant, intermediates, and product were obtained by calculating their phonon density of states, as depicted in Eq. 1 : 
    G=E+ZPE+kT∫F(ω)ln [1-exp(-ℏω/kT)]dω
 (1) where E is the energy, ZPE is the zero-point energy, the term \(kT\int F(\omega ){{{{\mathrm{ln}}}}}[1-\exp (-\frac{\hslash \omega }{kT})]d\omega\) was the correction of Gibbs free energy via thermodynamic analysis.